Rapid submarine ice melting in the grounding zones of ice shelves in West Antarctica Enhanced submarine ice-shelf melting strongly controls ice loss in the Amundsen Sea embayment (ASE) of West Antarctica, but its magnitude is not well known in the critical grounding zones of the ASE’s major glaciers. Here we directly quantify bottom ice losses along tens of kilometres with airborne radar sounding of the Dotson and Crosson ice shelves, which buttress the rapidly changing Smith, Pope and Kohler glaciers. Melting in the grounding zones is found to be much higher than steady-state levels, removing 300–490 m of solid ice between 2002 and 2009 beneath the retreating Smith Glacier. The vigorous, unbalanced melting supports the hypothesis that a significant increase in ocean heat influx into ASE sub-ice-shelf cavities took place in the mid-2000s. The synchronous but diverse evolutions of these glaciers illustrate how combinations of oceanography and topography modulate rapid submarine melting to hasten mass loss and glacier retreat from West Antarctica. The Amundsen Sea embayment (ASE) continues to be the region with the largest net mass loss in Antarctica [1] , [2] , and some of the highest rates of ice-shelf bottom melting [3] , [4] . Evidence suggests that increased circulation of warm and salty Circumpolar Deep Water (CDW) in the cavities underneath the ice shelves is a main trigger of, and contributor to, ice loss in the region [5] , [6] , [7] . The increased inflow of ocean heat and enhanced bottom ice melting in the cavities thins the ice shelves, contributing to grounding line retreat and weakening the contact with underlying bedrock, side margins, stabilizing ridges and pinning points such as ice rises. Consequently, the buttressing that the ice shelves afford their tributary glaciers diminishes causing the glaciers to accelerate and thin further, especially if the enhanced melting is concentrated near the grounding line [8] , [9] , [10] . Pine Island (PIG) and Thwaites (TG) glaciers, the two largest in the ASE, merited much attention due to their present and possible future large contributions to sea level rise [11] , [12] , [13] . Yet, some of the most rapid changes in the region are being observed in the Dotson and Crosson ice shelves ( Fig. 1a,b ) and their main tributary glaciers of Smith (SG), Pope (PG) and Kohler (KG). SG underwent the farthest grounding line retreat in the region of 35 km between 1996 and 2011 (ref. 13 ), Crosson Ice Shelf exhibited the largest average thickness loss between 1994 and 2012 (ref. 14 ), and grounded ice surfaces lowered by rates reaching 7 m per year in the period 2002–2010 ( Fig. 1c ; refs 1 and 15 ). The ice discharge of SG increased faster than those of PIG or TG between the mid 1990s and 2012 as its flow at the grounding line accelerated from 0.7 to 1.15 km per year (ref. 16 ). The flow speed of PG in the same period increased from 0.55 to 0.75 km per year, and that of KG from 0.8 to 1.1 km per year (ref. 16 ). 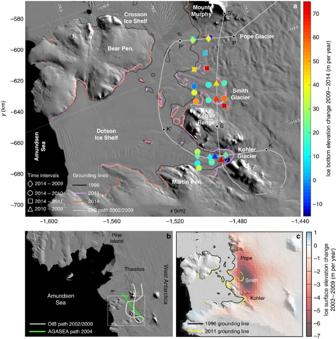Figure 1: The study area of the Dotson and Crosson ice shelves and their tributary glaciers. (a) The repeat flight path of the 2002 and 2009 Operation IceBridge (OIB) campaigns, with the letters S-S′, P-P′ and K-K′ marking the endpoints of the profiles inFigs 2,3,4. Colour scale shows bottom ice elevation changes at crossover locations of non-repeating OIB tracks between the years 2009 and 2014. At each crossover location, the bottom elevation of the earlier year is subtracted from that of the latter, hence positive values indicate bottom ice loss. The differences found are then averaged over the length of the time interval to facilitate comparisons. Uncertainty varies between∼35 m per year for the 1-year interval to∼7 m per year for the 5-year interval (Methods). Grounding lines are from refs13and19, and background image is from the 2008–2009 MODIS Mosaic of Antarctica50(MOA). (b) The study area ofFig. 1alocated on a map of the ASE region by the white rectangle showing the flight paths analysed here of the 2002 and 2009 OIB campaigns, and the 2004 AGASEA campaign along the Smith-Kohler glacier trunk. (c) Surface lowering rates for the period 2003–2009 adapted from ref.1. The authors used ICESat-1 measurements with the necessary corrections, with ATM and other data products applied as additional constraints to the surface shape and elevation time series. Figure 1: The study area of the Dotson and Crosson ice shelves and their tributary glaciers. ( a ) The repeat flight path of the 2002 and 2009 Operation IceBridge (OIB) campaigns, with the letters S-S′, P-P′ and K-K′ marking the endpoints of the profiles in Figs 2 , 3 , 4 . Colour scale shows bottom ice elevation changes at crossover locations of non-repeating OIB tracks between the years 2009 and 2014. At each crossover location, the bottom elevation of the earlier year is subtracted from that of the latter, hence positive values indicate bottom ice loss. The differences found are then averaged over the length of the time interval to facilitate comparisons. Uncertainty varies between ∼ 35 m per year for the 1-year interval to ∼ 7 m per year for the 5-year interval (Methods). Grounding lines are from refs 13 and 19 , and background image is from the 2008–2009 MODIS Mosaic of Antarctica [50] (MOA). ( b ) The study area of Fig. 1a located on a map of the ASE region by the white rectangle showing the flight paths analysed here of the 2002 and 2009 OIB campaigns, and the 2004 AGASEA campaign along the Smith-Kohler glacier trunk. ( c ) Surface lowering rates for the period 2003–2009 adapted from ref. 1 . The authors used ICESat-1 measurements with the necessary corrections, with ATM and other data products applied as additional constraints to the surface shape and elevation time series. Full size image Here we use airborne radar sounding to measure directly submarine ice loss in the grounding zones of the three main tributary glaciers of Dotson and Crosson ice shelves. NASA’s airborne Operation IceBridge (OIB) surveyed these areas in 2009 along a trajectory that was first overflown as part of an earlier campaign in 2002 ( Fig. 1a ). Subsequent OIB coverage of the area between 2009 and 2014 was along non-repeating lines, but provided several crossover points ( Fig. 1a ) that help assess changes post 2009, albeit at a less refined spatial resolution. Temporally, the period 2002–2009 spans the time of the fastest increase in three decades in mass loss from the study area and the ASE as a whole, while the years 2009–2014 coincide with a marked slowing down in the increase in the loss [1] , [11] , [15] , [16] . Spatially, the observations give a detailed view of the critical grounding zones compared with, and fill the gap between, the previous large-scale studies cited above that considered either grounded ice or floating ice shelves at coarser resolutions. The concurrent observations from three glaciers, furthermore, allow the examination of variations in melting rates, bed topographies and grounding line dynamics under similar glaciological and oceanic conditions. We find melting rates in the grounding zones of the three glaciers to be much higher than steady-state levels, removing as much as 300–490 m between 2002 and 2009 in the case of Smith Glacier (40–70 m per year). The intense unbalanced melting supports the hypothesis that a large increase in ocean heat influx into the sub-ice-shelf cavities of the ASE occurred in the mid-2000s. Averaged melting rates between 2009 and 2014 are similar or lower, which also is consistent with the slower increases in mass loss observed regionally by the end of the 2000s. Nonetheless, while Pope and Kohler glaciers stabilized, the grounding line retreat of Smith persisted. We attribute the different evolution of Smith Glacier to the retreat of its grounding line deeper allowing warmer waters to flood its grounding zone, and increasing ocean thermal forcing due to the lowering of the in situ melting point; as well as to the exposure of the glacier bottom to ocean water as the grounding line retreated rapidly. In contrast, Pope and Kohler had retreated to shallower terrain. Such combinations of ocean conditions and topography sustaining high submarine melting can hasten mass loss from West Antarctica. Furthermore, with ice bottom melting rates in the ASE already as high as we find here, radar sounding emerges as an effective observational tool for measuring those rates at high spatial resolution on continental scales, particularly in the grounding zones of rapidly retreating glaciers. Direct ice-shelf bottom measurements with radar sounding The radar sounding observations presented here have the significance of being direct measurements of the magnitude of bottom ice elevation changes in an Antarctic grounding zone. These direct measurements reflect the rate of basal melting once the contributions to total ice thinning of surface mass balance and dynamic changes are constrained, as discussed below. Magnitudes of ice-shelf thinning in the ASE are so large that they reach well above the 10–35 m vertical measurement uncertainty of the radar (Methods). The measurements are direct in the sense that they do not require the assumption of ice being in hydrostatic equilibrium as is the case of the methods usually applied to infer bottom melting rates [3] , [4] . The assumption of hydrostatic equilibrium is not valid in the grounding zones as ice actually lies lower than the equilibrium level over several kilometres downstream from the grounding line [17] . Ice shelves can also depart from hydrostatic equilibrium by grounding on bathymetric features as in the case of KG described below. Contributions of surface processes and dynamic thinning Total ice thinning is the sum of the observed changes in the top and bottom ice-shelf surface elevations. To isolate the thinning component that is due to bottom melting we seek to constrain the contributions of surface processes and of dynamic thinning. We constrain the former from repeat ATM measurements of grounded, slow moving ice areas. Such areas in the study region are Mount Murphy around longitude −111° and the Kohler Range around −113.5° and −115° ( Fig. 1a ). Between the years 2002 and 2009 the surface there lowered by 3–5 m (0.4–0.7 m per year; Fig. 2a ; Supplementary Fig. 1 ). These areas are located at altitudes that are between 300 and 600 m higher than the top surfaces of the grounding zones of the three glaciers ( Supplementary Fig. 1 ). The altitude difference means that the influences of temperature, accumulation rate and other factors on surface elevation change due to surface processes might not be the same at the lower altitude. ICESat-1 laser altimetry of the study area in the period 2003–2007 show that grounded, slow flowing areas changed little or thickened [18] , which suggests that the 3–5 m lowering we observe here is an upper limit on the contribution of surface processes to the thinning in the grounding zones. Surface lowering rates of fast moving, grounded ice directly upstream from the grounding lines reflect the combined contributions of surface processes and dynamic thinning. Use of these rates is supported by the similarity of flow speed gradients upstream and downstream of the grounding lines [16] . ATM data show surface lowering in the along-flow profiles of PG and KG of 25–30 m between 2002 and 2009 ( Figs 3a and 4a ), or ∼ 4 m per year. In the case of SG, Fig. 1c shows a maximum surface lowering of 7 m per year. The surface lowering signal of grounded, fast-moving ice therefore appears to be dominated by dynamic thinning with surface processes the smaller component. The combined contributions of dynamic thinning and surface processes therefore are roughly 10–15% of the observed ice-shelf thinning. This percentage, which is by coincidence close to the ratio of ice-shelf freeboard to its draft, means that the observed bottom ice loss is numerically similar to bottom melting. In what follows, we focus on changes at the ice-ocean interface, and use the terms bottom ice loss and out-of-balance bottom melting interchangeably. 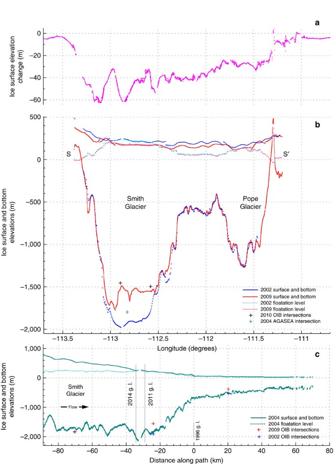Figure 2: Smith Glacier radar transects showing basal ice loss and corresponding surface elevation change between the years 2002 and 2009. (a) Surface elevation change between 2002 and 2009 as measured by ATM laser altimetry on the across-flow Smith Glacier (SG) transect delimited by S-S′ shown inFig. 1a. (b) The 2002 and 2009 ice surface and bottom MCoRDS profiles of SG along the transect delimited by S-S′ inFig. 1a. The hydrostatic floatation levels were found by taking freeboard elevation to be 0.12 of ice thickness, which was inferred from floating ice inFigs 3band4b; and taking sea surface to be at −33.9 m relative to the WGS84 ellipsoid, which was found from ATM 2009 measurements of ocean surface height in front of the Dotson Ice Shelf. The 2002 ice bottom appears partially dotted at some locations due to the lower density of available measurements there. (c) Ice surface and bottom along-flow profiles following the entire 2004 AGASEA trajectory shown inFig. 1b. In this and subsequent figures the vertical grey lines mark grounding line locations. The 1996 grounding line location is taken as the origin of thexaxis representing the distance along the flight path, and is indicated by a shorter grey line when bed topography is not available at its location. Figure 2: Smith Glacier radar transects showing basal ice loss and corresponding surface elevation change between the years 2002 and 2009. ( a ) Surface elevation change between 2002 and 2009 as measured by ATM laser altimetry on the across-flow Smith Glacier (SG) transect delimited by S-S′ shown in Fig. 1a . ( b ) The 2002 and 2009 ice surface and bottom MCoRDS profiles of SG along the transect delimited by S-S′ in Fig. 1a . The hydrostatic floatation levels were found by taking freeboard elevation to be 0.12 of ice thickness, which was inferred from floating ice in Figs 3b and 4b ; and taking sea surface to be at −33.9 m relative to the WGS84 ellipsoid, which was found from ATM 2009 measurements of ocean surface height in front of the Dotson Ice Shelf. The 2002 ice bottom appears partially dotted at some locations due to the lower density of available measurements there. ( c ) Ice surface and bottom along-flow profiles following the entire 2004 AGASEA trajectory shown in Fig. 1b . In this and subsequent figures the vertical grey lines mark grounding line locations. The 1996 grounding line location is taken as the origin of the x axis representing the distance along the flight path, and is indicated by a shorter grey line when bed topography is not available at its location. 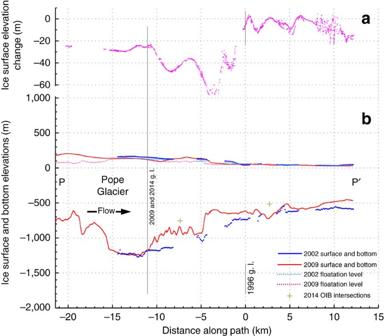Figure 3: Pope Glacier radar transects showing basal ice losses and corresponding surface elevation changes between the years 2002 and 2009. (a) Surface elevation change between 2002 and 2009 as measured by ATM laser altimetry on the along-flow Pope Glacier (PG) transect delimited by P-P′ shown inFig. 1a. (b) The 2002 and 2009 ice surface and bottom MCoRDS profiles of PG along the transect delimited by P-P′ inFig. 1a. The hydrostatic floatation levels were found as described in the caption ofFig. 2b. Full size image Figure 3: Pope Glacier radar transects showing basal ice losses and corresponding surface elevation changes between the years 2002 and 2009. ( a ) Surface elevation change between 2002 and 2009 as measured by ATM laser altimetry on the along-flow Pope Glacier (PG) transect delimited by P-P′ shown in Fig. 1a . ( b ) The 2002 and 2009 ice surface and bottom MCoRDS profiles of PG along the transect delimited by P-P′ in Fig. 1a . The hydrostatic floatation levels were found as described in the caption of Fig. 2b . 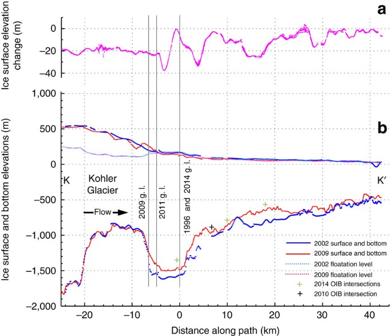Figure 4: Kohler Glacier radar transects showing basal ice losses and corresponding surface elevation changes between the years 2002 and 2009. (a) Surface elevation change between 2002 and 2009 as measured by ATM laser altimetry on the along-flow Kohler Glacier (KG) transect delimited by K-K′ shown inFig. 1a. (b) The 2002 and 2009 ice surface and bottom MCoRDS profiles of KG along the transect delimited by K-K′ inFig. 1a. The hydrostatic floatation levels were found as described in the caption ofFig. 2b. Full size image Figure 4: Kohler Glacier radar transects showing basal ice losses and corresponding surface elevation changes between the years 2002 and 2009. ( a ) Surface elevation change between 2002 and 2009 as measured by ATM laser altimetry on the along-flow Kohler Glacier (KG) transect delimited by K-K′ shown in Fig. 1a . ( b ) The 2002 and 2009 ice surface and bottom MCoRDS profiles of KG along the transect delimited by K-K′ in Fig. 1a . The hydrostatic floatation levels were found as described in the caption of Fig. 2b . Full size image Rapid bottom ice loss in the grounding zones The ice loss in the SG grounding zone between 2002 and 2009 was intense. In that period, the MCoRDS radar sounding data show that the glacier lost 300 to 490 m in draft thickness in the part of the across-flow transect between longitudes −113.05° and −112.50° ( Fig. 2b ), representing an average rate of 40 to 70 m per year depending on location. The coincident ATM laser altimetry measured freeboard surface lowering of 30–60 m ( Fig. 2a ) in 2002–2009 (4.3–8.6 m per year). The inferred hydrostatic floatation levels indicate that this part of SG was nearly or already floating in 2002 ( Fig. 2b ), and certainly floating in 2009 after thinning. With the ice being afloat, the surface lowering numbers therefore corroborate the thinning observed by the radar sounding. The thinning in 7 years represents 22% of the ice thickness at −112.88° ( Fig. 2b ). A location of similarly high thinning, shown by both radar sounding and surface altimetry, is the western margin of the glacier at −113.05° ( Fig. 2a,b ). In the period 2009–2014, high rates of bottom ice loss persisted in the innermost and deeper part of the cavity ( Fig. 1a ; Supplementary Fig. 2 ; Supplementary Table 1 ). PG also shows extensive thinning and surface lowering, especially upstream from the 1996 grounding line location ( Fig. 3a,b ). Bottom ice loss in places reaches 200–250 m over the 2002–2009 period (29–36 m per year). There is spatial correspondence between the changes in ice thickness from MCoRDS and ATM surface lowering extents ( Fig. 3a ). In the period 2009–2014 the bottom ice loss rates were similar at two points on the 2002/2009 transect, and lower at two other points off that transect ( Fig. 1a ; Supplementary Fig. 2 ; Supplementary Table 1 ). The grounding line retreat of PG could not be quantified previously, but the observations here show (Methods) that it retreated by 11 km between 1996 and 2009 ( Fig. 3b ), which is supported by recent findings [19] . The profile of KG ( Fig. 4b ) shows the floating ice-shelf downstream from kilometre 11 to have thinned by 100–200 m between 2002 and 2009 (14–29 m per year), and that the surface lowered correspondingly ( Fig. 4a ). In the period 2009–2014, those rates persisted ( Fig. 1a ; Supplementary Fig. 2 ; Supplementary Table 1 ), except for one anomalous measurement of higher bottom ice loss. The 2002–2009 transect ( Fig. 4b ) shows that bottom ice loss in the grounding zone has no corresponding surface lowering between kilometres 0 and −2. This is a consequence of the glacier not being in hydrostatic equilibrium as KG exhibits a more complex grounding zone. The glacier is grounded between kilometres 0 and 1 ( Fig. 4b ), upstream of which ocean is present and enhanced melting has occurred, before being grounded again around kilometre −8 in 2009 ( Fig. 5 ). These observations add to the inventory of kilometre-long grounding zones over which the extent of contact between ice, bed and ocean water vary spatially [17] , [20] , [21] . 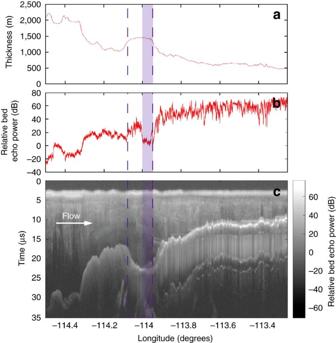Figure 5: Radar sounding data show evidence of an isolated area of grounding between two floating portions of the Kohler Glacier grounding zone. (a) Across a region of nearly constant ice thickness (dashed magenta lines), (b) the approximately 20 dB drop in relative bed echo power is consistent with a basal interface transition from ocean water to bedrock44,45indicating that the glacier is grounded in the part of the profile delimited by the magenta rectangle. (c) A 2009 MCoRDS radargram of the Kohler Glacier grounding zone. Figure 5: Radar sounding data show evidence of an isolated area of grounding between two floating portions of the Kohler Glacier grounding zone. ( a ) Across a region of nearly constant ice thickness (dashed magenta lines), ( b ) the approximately 20 dB drop in relative bed echo power is consistent with a basal interface transition from ocean water to bedrock [44] , [45] indicating that the glacier is grounded in the part of the profile delimited by the magenta rectangle. ( c ) A 2009 MCoRDS radargram of the Kohler Glacier grounding zone. Full size image The observed high rates of ice-shelf thinning reflect out-of-balance melting. Spatially averaged steady-state melting for the Dotson–Crosson ice shelves were estimated to be roughly 9.5 m per year (ref. 3 ) and 7.8–11.9 m per year (ref. 4 ). Melting rates specifically in the grounding zones of the two ice shelves were calculated to be 12–20 m per year, with double those values occurring 10–15 km farther downstream [4] . The large difference between the estimated steady-state melting rates and the rates observed here demonstrates the intensity of out-of-balance melting concentrated in the grounding zone, particularly of SG. The high rates of bottom melting observed here strongly suggest that the Dotson and Crosson sub-ice-shelf cavities experienced a larger influx of ocean heat sometime between 2002 and 2009. Such influx accords with the increase in mass loss from all of the ASE major glaciers in the mid-2000s, including the tributaries of the Dotson and Crosson ice shelves [1] , [11] , [16] . It also accords with the higher observed thinning rates of ASE ice shelves outside their grounding zones, including Crosson and PIG, during the mid-2000s compared with earlier years [14] . A regional scale, simultaneous change is most likely the result of increased temperature and/or flow of warm waters in the sub-ice-shelf cavities. Warm modified CDW was observed to flow southward [22] , [23] in a trough in the continental shelf off the Dotson Ice Shelf [24] . It is not yet known whether the trough continues to the grounding zone unhindered by ridges, or whether warm waters could also reach the Dotson–Crosson grounding zones through the Crosson sub-ice-shelf cavity. A large number of ice rises in the Dotson Ice Shelf, especially between the Kohler Range and Bear Peninsula ( Fig. 1a ), suggests that its cavity away from the grounding zone might be shallow and/or traversed by a ridge there hence limiting the access of deep warm waters. The increases in ice flow speeds and volume discharge of the three glaciers, and in mass loss from the ASE region as a whole, slowed by 2009 or 2010 (refs 1 , 11 and 16 ). Again, the regional scale of the slowing suggests widespread changes in oceanic conditions on the continental shelf leading to slower increases in the influx of ocean heat. Such changes in ocean conditions in the vicinity of PIG between 2010 and 2012 were associated with a decrease in its bottom melting [7] , and our results suggest similar changes in the Dotson–Crosson area. Thus, the measured bottom ice loss rates in the period 2009–2014 are either similar to, or lower than, those in 2002–2009 ( Fig. 1a ; Supplementary Fig. 2 ; Supplementary Table 1 ). These rates indicate that the influx of ocean heat might have started to stabilize around 2009, and that the observed changes in the areas of Dotson–Crosson and PIG were part of a widespread event. Oceanic conditions and melting rates beneath the Dotson–Crosson ice shelves driven by CDW variability could be modulated by changes in the extent of a large winter polynya, which opens off the Dotson Ice Shelf and Bear Peninsula [25] . Dense polynya water at the surface melting temperature, resulting from sea ice formation and the accompanying brine rejection and loss of buoyancy, was hypothesized to influence submarine melting rates by mixing and modifying water properties in sub-ice-shelf cavities [26] , [27] . A decrease in the extent of winter polynyas could therefore reduce the volume of the dense, cold water available to mix with warm CDW at depth hence contributing to enhanced bottom melting and vice versa. SG experienced the highest melting rates in 2002–2009 and the farthest grounding line retreat by 2011. Unlike the other two glaciers, its rapid melting persisted in 2009–2014, and it continued to retreat between 2011 and 2014, albeit at a slightly slower pace. We explain these differences by a combination of cavity oceanic conditions and bed topography. SG has retreated enough to reach a 2,000-m deep trench [28] after having been grounded at 500–800 m depth in 1996 (ref. 13 ). This retreat has created a topographic feature having the shape of an elongated bowl that is more than a kilometre deep from rim to bottom ( Fig. 3f in Rignot et al . [13] ). We propose that the deepening and the bed topography uncovered by the retreat are favourable to giving access to warm dense water in the SG grounding zone contributing to its rapid melting and retreat, in a manner similar to the hypothesized flooding of the Jakobshavn cavity with warm water that passed over a sill at the mouth of its fjord [29] . Available evidence suggests that the temperature of the denser water reaching the deepening SG grounding zone would be higher. Thus, water temperature and salinity profiles from the vicinity of PIG show that the densest water at 1,000 m depth is ∼ 1 °C warmer than that at 500 m (refs 6 and 7 ). Furthermore, the relationship between deeper grounding lines and higher bottom melting was previously noted [9] , [28] , [30] . The three glaciers have in common the great depths of their grounding lines ( Figs 2c , 3b and 4b ), but the deepest by far is SG which in 2014 is grounded at nearly 2,100 m below sea level. As the melting point of seawater decreases with depth at a rate of 0.75 °C km −1 (ref. 31 ), the SG grounding line corresponds to an additional ∼ 0.8 °C of ocean thermal forcing compared with PIG, of which the grounding line is at 1,000 m depth [5] . We further hypothesize that the rapid retreat of the SG grounding line could explain at least part of the observed high bottom melting rates. Such fast retreat transforms the basal boundary condition of grounded ice from contact with bed to exposure to ocean water and much higher melting [32] . Rapid thinning will hence result if the glacier cannot adjust quickly enough to compensate mass lost to the ocean at the newly exposed bottom surface. SG retreat will probably slow given that its bed upstream from the 2014 grounding line rises inland over ∼ 10 km, and its upper surface starts rising above the flotation level ( Fig. 2c ). The grounding lines of Kohler and Pope glaciers did not retreat as deeply ( Figs 3b and 4b ), hence their grounding zones were not as susceptible to the increased inflow of warmer waters as that of SG. KG is the glacier with the smallest grounding line retreat between 1996 and 2014 and relatively the lowest bottom melting between 2002 and 2009. Its bed rises steeply by 300 m over <1.5 km directly upstream from the 2009 grounding line and its upper surface rises well above floatation level ( Fig. 4b ). Later, under the hypothesized change in oceanic conditions around 2009, such bed and surface geometry contributed to the grounding line actually readvancing between 2009 and 2011 and again between 2011 and 2014. PG has the second farthest grounding line retreat by 2014 and second largest bottom melting between 2002 and 2009. Its bed rises inland, but more gently than KG, and its 2009 grounding line is still ∼ 5 km downstream of the first prominent bed topographic rise located upstream from kilometre −16 ( Fig. 3b ). It also exhibits an ice plain (characterized by an upper surface having low slope and at or only slightly above floatation level [33] ) extending over several kilometres. These geometric factors probably contributed to the 2014 PG grounding line maintaining its 2009 location, or regaining it after an intervening retreat, under the modified oceanic conditions. Observations such as those presented here can contribute to more rigorous explorations of the differences in behaviour among the rapidly changing glaciers of Antarctica and their possible evolutions, and the geometric and dynamic factors involved [5] , [10] , [34] . This requires knowledge of ocean forcing changes and 3D modelling of the coupled glacier/ice-shelf/ocean system, including accurate sub-ice shelf bathymetry, an evolving ice-shelf bottom morphology, cavity circulation and bed topography [35] , [36] , [37] . Concerning the ASE more specifically, the observations are a compelling illustration of the changes that the ASE region is experiencing as it continues to be the largest source of Antarctic mass loss to the ocean. Radar sounding offers an unprecedented view of the actual bottom ice loss over wide areas in the critical grounding zones of ice shelves. Measuring ice thinning is difficult in grounding zones experiencing not only rapid melting but also changing geometry and location as grounding lines migrate. Migration reconfigures continuously the floatation conditions in and around a grounding zone, and changes the location and extent of grounding on ridges and ice rises, hence affecting the accuracy of bottom melting estimates based on ice surface heights. At the same time, submarine ice losses in these rapidly changing areas are so large that they can now be measured directly with airborne radar sounding. This makes possible a new approach for the monitoring of ice-shelf thickness changes on regional or continental scales as they respond to thermal forcing variability of the ocean and more generally to climate change. MCoRDS and HiCARS radar sounding We use the Level-2 Multichannel Coherent Radar Depth Sounder [38] (MCoRDS) airborne measurements to trace glacier bottom profiles. Data have an along-track resolution of ∼ 25 m and depth resolution of ∼ 18 m. Across-track spatial resolution varies with aircraft height, surface roughness and ice thickness between 641 and 5,416 m. Pre-OIB and OIB airborne campaigns surveyed along the path shown in Fig. 1a in 2002 and again in 2009, respectively, which allowed the comparisons of extended glacier transects ( Figs 2b , 3b and 4b ). When comparing these transects, only points that are closer than 200 m in the horizontal are considered. We impose this restriction to minimize the effects of ice bottom slope on the change signal where tracks do not repeat exactly. Post-2009 ice bottom changes ( Fig. 1a ) are found from crossover analyses of OIB tracks from 2009, 2010, 2011 and 2014. The post-2009 tracks, which were flown in grids, are not shown here, but can be viewed on the Web with the IceBridge Planning Data Tool ( icebridge.sr.unh.edu/icebridge/ant/ ). We analyse crossovers at the points where tracks from the years 2010 and 2014 intersect with the 2002/2009 path, and at other points in the grounding zones where tracks from 2010 and 2011 intersect with those from 2014. Measurements by a system similar to MCoRDS flying at low altitude, and by MCoRDS itself at high altitude, suggest a vertical uncertainty of ±10 m when the ice bottom is detected [39] , [40] . We find here an indication of data consistency from two crossover locations at Pope and Kohler glaciers ( Fig. 1a ), where for the 2009 data the difference in measured ice bottom elevations is 26 and 12 m, respectively. Taking a conservative measurement uncertainty of 25 m, the uncertainty when comparing soundings from two different years is 35 m. When expressing bottom elevation change as a yearly average the uncertainty is divided by the number of years separating the two measurements. Hence, for the post-2009 crossover estimates ( Fig. 1a ), the uncertainty varies between ∼ 35 m per year for the 1-year interval to ∼ 7 m per year for the 5-year interval. The SG ice thickness transect along its trunk ( Fig. 1b ) is from the 2004 Airborne Geophysical Survey of the Amundsen embayment [41] (AGASEA) that used the Hi-Capability Radar Sounder (HiCARS). The uncertainty of HiCARS elevation measurements is 72 m (ref. 41 ). Neither data set makes assumptions about a firn layer. Radar sounding was used previously to measure bottom ice loss in Greenland [42] , and in situ bottom melting in Antarctica was measured with phase-sensitive radar [32] , [43] . In addition to bottom elevations, radar sounding echograms can in some cases be used to determine whether ice bottoms are underlain by water or bedrock, hence locating where the ice might be floating or grounded. The method relies on reflected radar signals being brighter at ice–water interfaces because of the higher contrast in dielectric properties across those interfaces compared with ice-bedrock ones [44] , [45] , and is described in Fig. 5 . We also used radar sounding profiles to locate grounding line locations. If the ice has thinned between the observations from 2002 and 2009, then the 2009 grounding line is at the first point moving upstream where the 2002 and 2009 glacier bottoms begin to coincide. ATM laser altimetry Surface elevation changes are from measurements by the Airborne Topographic Mapper (ATM) laser altimeter that has been flying since 2009 as part of OIB and had flown over Antarctica earlier during the years 2002, 2004 and 2008. ATM measurements were acquired coincidentally with the MCoRDS soundings during the surveys of 2002 and 2009, hence providing independent corroboration of the thinning observed by radar sounding. The data (Level-2 Icessn Elevation, Slope, and Roughness data) have an along-track spacing of 50 m (ref. 46 ). Our algorithm to find surface elevation changes between repeat ATM observations [47] considers only points within 25 m from each other. The uncertainty of ATM measurements on grounded ice is assessed to be less than 9 cm (ref. 46 ). On floating ice, further uncertainty is added by RMS tidal heights in the ASE of 40–60 cm (ref. 48 ). Grounding line locations The 1996 and 2011 grounding line locations were found by applying differential satellite synthetic‐aperture radar interferometry [13] , [49] to data from the Earth remote sensing satellites 1 and 2 (ERS-1 and 2). The 2014 grounding lines were similarly found from Sentinel-1 data [19] . Estimated spatial accuracy of grounding line locations is ±100 m. We use the term ‘grounding zones’ to refer to the vicinity of the grounding lines. Data availability The MCoRDS and HiCARS radar sounding data, and ATM Lidar data, that support the findings of this study were collected during Operation IceBridge and earlier airborne campaigns and are available from the NASA Distributed Active Archive Center (DAAC) at The National Snow and Ice Data Center (NSIDC), https://nsidc.org/data/icebridge/data_summaries.html . How to cite this article: Khazendar, A. et al . Rapid submarine ice melting in the grounding zones of ice shelves in West Antarctica. Nat. Commun. 7, 13243 doi: 10.1038/ncomms13243 (2016). Publisher's note: Springer Nature remains neutral with regard to jurisdictional claims in published maps and institutional affiliations.